Intrinsic measurements of exciton transport in photovoltaic cells Organic photovoltaic cells are partiuclarly sensitive to exciton harvesting and are thus, a useful platform for the characterization of exciton diffusion. While device photocurrent spectroscopy can be used to extract the exciton diffusion length, this method is frequently limited by unknown interfacial recombination losses. We resolve this limitation and demonstrate a general, device-based photocurrent-ratio measurement to extract the intrinsic diffusion length. Since interfacial losses are not active layer specific, a ratio of the donor- and acceptor-material internal quantum efficiencies cancels this quantity. We further show that this measurement permits extraction of additional device-relevant information regarding exciton relaxation and charge separation processes. The generality of this method is demonstrated by measuring exciton transport for both luminescent and dark materials, as well as for small molecule and polymer active materials and semiconductor quantum dots. Thus, we demonstrate a broadly applicable device-based methodology to probe the intrinsic active material exciton diffusion length. Excitons are Coulombically-bound electron-hole pairs that serve as energetic intermediates in semiconductors. In many emerging semiconductor materials, the exciton and its properties feature prominently in determining device applications due to large binding energies that stabilize the exciton against thermally-driven dissociation [1] , [2] , [3] , [4] , [5] , [6] , [7] , [8] . Indeed, the high stability of the exciton has driven much research into the design of active materials and device architectures for organic light-emitting devices and organic photovoltaic cells (OPVs) [9] , [10] , [11] , [12] , [13] , [14] , [15] . Recently, there has also been growing interest in manipulating exciton transport at semiconductor heterointerfaces for devices like excitonic transistors [16] , [17] , [18] . For OPVs, in particular, excitons must migrate to a dissociating electron donor–acceptor (D-A) interface, making exciton transport a critical step towards efficient photoconversion [19] , [20] , [21] , [22] , [23] , [24] . Consequently, substantial previous work has been directed at both the measurement and engineering of the exciton diffusion length ( L D ). These efforts are essential as the scale of L D dictates the optimal active layer thickness and domain size of D–A blends in planar (PHJ) and bulk heterojunction (BHJ) OPVs, respectively [25] , [26] , [27] , [28] , [29] . Probing exciton migration often relies on tracking the end-of-life products of excitons, including photons from exciton recombination and charge carriers from exciton dissociation [30] , [31] . For luminescent materials, L D can be determined from a steady-state or time-resolved photoluminescence (PL)-based measurement [22] , [32] , [33] . Emitted photons reflect excitons that fail to reach the dissociating interface. While capable of yielding a materials-relevant value of L D , this method is only sensitive to diffusive states that can decay radiatively and therefore cannot be applied to materials forming weakly emissive or dark excitons [34] , [35] , [36] . Since many high-performing active materials are weakly luminescent or dark [7] , [12] , [35] , [37] , [38] , it is essential to develop more general means to accurately probe exciton transport in working devices. A more general approach to extract L D is by fitting the measured photocurrent (i.e., external quantum efficiency) spectrum of a bilayer OPV [39] , [40] , [41] . Device-based methods are attractive as they probe the L D in a practical environment, as opposed to the often idealized structures utilized for PL measurements. This method is equally applicable to all excitons regardless of photoluminescence efficiency. Photoconversion can be considered in terms of four component processes, each with its own efficiency, namely light absorption ( η A ), exciton diffusion and dissociation ( η D ), charge transfer (CT) state separation ( η CS ), and free carrier collection ( η FC ). As such, with knowledge of η CS and η FC , coupled with an optical transfer matrix model for η A , η D and L D can be extracted by fitting with a diffusion equation. In practice, the values of η CS and η FC are not known, and frequently taken as unity or assumed to be fixed with changes in device architecture [39] , [42] , [43] , [44] , [45] . Thus, the extracted value of L D is a lower bound to the actual, materials-specific L D . This limitation, coming from unknown geminate and non-geminate recombination losses, must be overcome in order to extract intrinsic, materials-specific values of L D . Recently, we reported a technique based on transient photovoltage to overcome the non-geminate recombination limitation on extracting L D from OPVs [46] , [47] . Photovoltage can be quantitatively translated into the number of free carriers stored within the device. For timescales much shorter than the carrier lifetime, the free carrier generation rate can be extracted from the initial photovoltage rise induced by illumination. The previously unknown η FC , therefore, can be quantitively measured by comparing the results of photovoltage and photocurrent measurements. Interestingly, η FC is found to be near-unity at short-circuit for many PHJ systems. Consequently, an inability to quantify geminate recombination loss is the primary factor frustrating accurate extraction of L D in devices. Despite the presence of unknown recombination losses, it is possible to measure the intrinsic L D from a device without the need to assume a value for η CS . Previously, Vandewal et al. have shown that relaxed interfacial CT states (lowest energy) are the dominant source for free carrier generation in a wide range of D–A systems [48] . This conclusion is further confirmed by recent work by Kurpiers et al. [49] . The value of η CS is thus independent of whether a carrier originates from the donor or acceptor exciton. As such, a ratio of the donor and acceptor internal quantum efficiencies ( η IQE ) cancels this unknown quantity and depends only on the exciton harvesting efficiencies ( η D ) at short-circuit: 
    η _IQE^D/η _IQE^A = η _D^Dη _CS/η _D^Aη _CS = η _D^D/η _D^A
 (1) In order to model η D , exciton diffusion is treated with a one-dimensional steady-state diffusion equation: 
    0 = D∂ ^2n( x )/∂ x^2 - n( x )D/L_D^2 + G( x ) - n( x )k_F with L_D = √(Dτ)
 (2) where n is the exciton density, D is the diffusion coefficient, τ is the exciton lifetime, and G is the optical exciton generation rate calculated by transfer matrix modeling. For systems with a spectral overlap of donor emission and acceptor absorption, the rate of donor–acceptor Förster energy transfer (rate constant: k F ) must be included. From the steady-state exciton density profile n ( x ), the η D can be determined as: 
    η _D = 1 - ∫n(x)/τdx/∫G( x )dx
 (3) By fitting the η D ratio in eq. ( 1 ) as a function of active layer thickness, L D values for the donor and acceptor materials can be extracted simultaneously. In this work, we apply the photocurrent-ratio method to extract L D for both luminescent and dark organic semiconductors, including both small molecule and polymer active materials. We further demonstrate the broad utility of this approach by also extracting L D for thin films of colloidal, inorganic semiconductor quantum dots. In order to compare the results of the photocurrent-ratio method to well-established photoluminescence quenching methods, we first consider the archetypical donor–acceptor pairing of boron subphthalocyanine chloride (SubPc) and C 60 (Fig. 1a ), where both active materials are luminescent. This system shows negligible non-geminate recombination loss at short-circuit [50] , [51] , and prior work suggests that free carriers are likely generated from a single relaxed CT state [52] , allowing eq. ( 1 ) to be applied. It is worth noting that in devices limited by non-geminate recombination, η FC can be measured using transient photovoltage, leading to a modified, but equally useful form of eq. ( 1 ). For this luminescent pairing, we demonstrate that the values of L D extracted using our device-based method are in excellent agreement with those extracted using conventional PL-based measurements. Importantly, we further show that our device-based method yields the intrinsic material L D even for devices that suffer from very low efficiency. Fig. 1 Device architectures and quantum efficiency spectra for SubPc-C 60 planar OPVs. a Molecular structure of SubPc and C 60 . b Device architecture for SubPc-C 60 planar OPVs. The SubPc thickness X varies from 10 nm to 45 nm. c Energy-level diagram for the devices in b . d The η EQE spectra measured at short-circuit as a function of SubPc layer thickness. e The η IQE spectra calculated by dividing the η EQE spectra in d by the η A calculated using a transfer matrix model. The extinction coefficients ( k ) of SubPc (purple dash line) and C 60 (brown dot line) are also shown Full size image Extracting L D from a ratio of internal quantum efficiencies To accurately measure L D in bilayer OPVs, it is important to ensure that the only mechanism for exciton dissociation is at the donor–acceptor interface. Quenching at other interfaces or via bulk-ionization will lead to errors in the extracted L D . 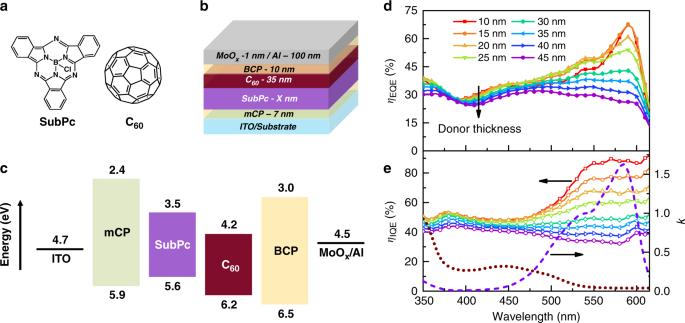Fig. 1 Device architectures and quantum efficiency spectra for SubPc-C60planar OPVs.aMolecular structure of SubPc and C60.bDevice architecture for SubPc-C60planar OPVs. The SubPc thickness X varies from 10 nm to 45 nm.cEnergy-level diagram for the devices inb.dTheηEQEspectra measured at short-circuit as a function of SubPc layer thickness.eTheηIQEspectra calculated by dividing theηEQEspectra indby theηAcalculated using a transfer matrix model. The extinction coefficients (k) of SubPc (purple dash line) and C60(brown dot line) are also shown Figure 1b shows the SubPc-C 60 PHJ OPV used for the measurement of L D . The wide energy gap organic semiconductors 1,3-bis(carbazol-9-yl)benzene (mCP) and bathocuproine (BCP) are employed as exciton blocking layers (EBLs) to prevent exciton quenching at active layer-electrode interfaces. The exclusion of quenching at the electrodes is critical for accurate measurements of L D as exciton loss is observed when SubPc is in direct contact with ITO or the commonly used buffer layer MoO x (Supplementary Figure 1 ) [53] . A 1-nm-thick layer of MoO x is used to increase the cathode work function and reduce the built-in electric field ( E bi ) to exclude efficient exciton bulk-ionization processes at short-circuit [54] . This is especially important for the SubPc-C 60 system since both materials have been observed to show efficient free carrier generation in Schottky OPVs [55] , [56] . While the application of a forward bias can also be used to reduce E bi , the resulting carrier injection into the device could lead to exciton quenching, and an underestimate of L D . It is worth noting that while a reduced E bi could hinder the separation of relaxed CT states at the donor–acceptor interface, we will demonstrate that this does not impact our measurement provided η CS is identical for charges originating from both active materials. Figure 1d shows external quantum efficiency ( η EQE ) spectra for SubPc-C 60 PHJ devices as a function of SubPc donor-layer thickness with the acceptor and buffer layer thicknesses held fixed. 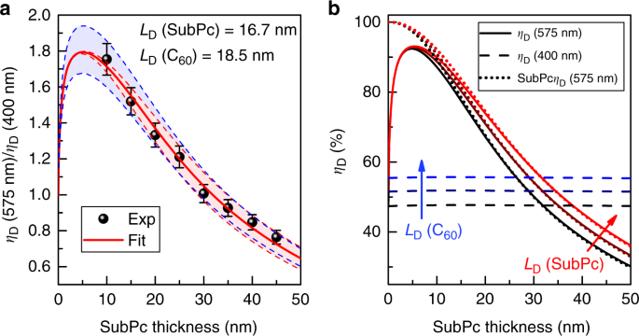Fig. 2 ExtractingLDfrom the thickness dependence of the diffusion efficiency ratio.aDiffusion efficiency ratio (λ= 575 nm toλ= 400 nm) as a function of SubPc layer thickness with the corresponding exciton diffusion length (LD) extracted from the fit (solid red line) to the data. Red (blue) dash lines are simulated diffusion efficiency ratio curves for a 10% change in extracted SubPc or C60LDwhile keeping the counterpartLDfixed. Error bars of diffusion efficiency ratio were determined based on the standard deviation of measured devices.bSolid lines are the diffusion efficiency atλ= 575 nm as a function of SubPc layer thickness for different SubPcLD( = 15.0/16.7/18.3 nm) and fixed C60LD= 18.5 nm. Similarly, the horizontal dash lines are the diffusion efficiency atλ= 400 nm for different C60LD( = 16.7/18.5/20.3 nm) and fixed SubPcLD= 16.7 nm. The diffusion efficiencies of SubPc atλ= 575 nm are also plotted as dot lines The η A of the active materials calculated using a transfer matrix formalism (Supplementary Figure 2 ) allows the η EQE spectra to be converted to η IQE spectra (Fig. 1e ) [41] . To ensure the accuracy of the simulated η A , the result from transfer matrix modeling is checked against experimentally determined device reflectivity (through the anode, reflecting off the cathode) measured at an incident angle of 15° to the substrate normal. 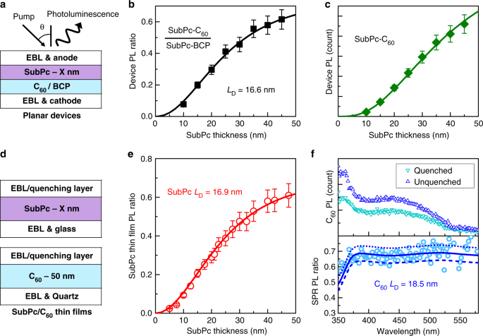Fig. 3 Photoluminescence-based measurements of exciton diffusion length.aOPVs used for the extraction ofLDvia photoluminescence (PL) quenching having the structure: ITO/7 nm mCP/X ( = 10–45) nm SubPc/35 nm C60(quenched) or BCP (unquenched)/10 nm BCP/1 nm MoOx/100 nm Al. The quenched samples are the same set of devices used for internal quantum efficiency measurements.bPL ratio defined in eq. (5) versus SubPc thickness.cSubPc PL intensity of the quenched samples versus SubPc thickness. The solid line is fit of the data using eq. (4). Error bars reflect the run-to-run variation in PL intensity (standard deviation).dArchitectures for conventional thin-film PL ratioLDmeasurements of SubPc and C60. SubPc architectures have the structure: glass/10 nm mCP/X ( = 5.0–47.5) nm SubPc/10 nm HATCN (quenched) or mCP (unquenched) while C60architectures have the structure: quartz/10 nm BCP/50 nm C60/10 nm HATCN (quenched) or BCP (unquenched).eThe PL ratio of SubPc films as a function of SubPc thickness.fExcitation spectra (upper panel) for the quenched and unquenched C60films at an emission wavelength of 750 nm. The resulting spectrally resolved (SPR) PL ratio versus pump wavelength is shown in lower panel. SubPc films and devices are all pumped withλ= 500 nm light. The incident angle is 70° for all incident light. Error bars for PL ratios are propagated from measured spectra and are proportional to the standard deviation in PL intensity measured multiple times The simulated 1-reflectivity ( R ) spectra (absorption of the device stack) agree well with experimental results as a function of donor thickness (Supplementary Figure 3 ). For the device with a donor thickness of 10 nm, the maximum η EQE (at λ = 590 nm, SubPc absorption) exceeds 65% and the corresponding η IQE is about 85%. This indicates that both exciton harvesting and charge collection are efficient in this device despite the reduced E bi . From the extinction coefficients (k) of SubPc and C 60 , spectral regions of dominant absorption for both donor and acceptor can be isolated. Accordingly, for the construction of the η IQE ratio, the individual η IQE of the donor and acceptor are extracted from λ = 575 nm (primarily SubPc absorption) and λ = 400 nm (primarily C 60 absorption), respectively. Consistent with eq. ( 1 ), a η D ratio ( λ = 575 nm to λ = 400 nm) is calculated as a function of SubPc thickness (Fig. 2a ), which will be fit for L D . Fig. 2 Extracting L D from the thickness dependence of the diffusion efficiency ratio. a Diffusion efficiency ratio ( λ = 575 nm to λ = 400 nm) as a function of SubPc layer thickness with the corresponding exciton diffusion length ( L D ) extracted from the fit (solid red line) to the data. Red (blue) dash lines are simulated diffusion efficiency ratio curves for a 10% change in extracted SubPc or C 60 L D while keeping the counterpart L D fixed. Error bars of diffusion efficiency ratio were determined based on the standard deviation of measured devices. b Solid lines are the diffusion efficiency at λ = 575 nm as a function of SubPc layer thickness for different SubPc L D ( = 15.0/16.7/18.3 nm) and fixed C 60 L D = 18.5 nm. Similarly, the horizontal dash lines are the diffusion efficiency at λ = 400 nm for different C 60 L D ( = 16.7/18.5/20.3 nm) and fixed SubPc L D = 16.7 nm. The diffusion efficiencies of SubPc at λ = 575 nm are also plotted as dot lines Full size image By fitting the η D ratios in Fig. 2a , we simultaneously extract L D values for SubPc and C 60 of L D = (16.7 ± 1.7) nm and L D = (18.5 ± 1.9) nm, respectively. Due to the spectral overlap of SubPc PL emission and C 60 absorption, donor–acceptor Förster energy transfer is included when using eq. ( 2 ). We have previously measured the SubPc-C 60 Förster radius ( R 0 ) to be 2.1 nm, consistent with the value of 2.1 nm calculated using Förster theory [32] . This value is short compared to the intrinsic L D of SubPc, and hence does not significantly impact our measurement of L D as diffusion is the dominant mechanism for harvesting in SubPc. As only the donor thickness is varied, the L D of the donor and acceptor have different roles in determining the overall behavior of the η D ratio as thickness changes (dash lines in Fig. 2a ). For example, if the SubPc L D is varied by 10% (C 60 L D fixed), the resulting η D ratios converge at small thickness while diverging at larger thickness, varying the shape of the dependence on thickness. Similar changes in the C 60 L D (10%, SubPc L D fixed) lead only to changes in the magnitude of the η D ratio leaving the shape unchanged. To show this more explicitly, the values of η D at λ = 575 nm and 400 nm are plotted as a function of donor thickness in Fig. 2b . The observation of a constant acceptor η D with increasing donor thickness offers some inherent advantages. First, the L D of the donor and acceptor can be fit independently, as the shape of the η D ratio (or normalized η D ratio) only depends on donor L D . As such, any non-ideality in acceptor L D measurement, such as exciton loss at the acceptor-cathode interface, would not reduce the accuracy of donor L D provided free carriers are still only generated at the D–A interface. In addition, the relative change in η CS with donor thickness is directly reflected by the acceptor η IQE . Accordingly, the decrease in η IQE (400 nm) with SubPc thickness (Fig. 1e ) indicates that a thicker donor layer leads to a lower η CS . This is likely due to an increase in bulk resistance of the donor layer that consumes more built-in voltage and thus reduces the electric field strength at D–A interface [57] . Photoluminescence-based L D measurements To determine whether the L D extracted from the η IQE ratio is intrinsic, conventional PL-based measurements are carried out for both SubPc and C 60 . In many previous studies, η EQE -based measurements of L D have not been in agreement with those extracted from PL due to geminate recombination losses [46] , [50] , which are in general not negligible. If the recombination limitations are fully overcome in the method described here, these measurements should yield the same L D . For luminescent SubPc, the intrinsic L D is extracted using thickness-dependent PL quenching and compared to the result obtained using the photocurrent-ratio method. In order to make a proper comparison, PL-quenching measurements are carried out on the identical device architecture used to measure L D via η IQE (Fig. 3a ). Light having a wavelength of λ = 500 nm is incident through the ITO anode at an angle θ of 70°. As the emitted photons represent the excitons that fail to reach D–A interface, the PL intensity can be expressed as: 
    PL = η _A(1 - η _D)(I_inη _PLη _det)
 (4) where I in is the incident photon flux, η PL is the photoluminescence efficiency, η det is the detection efficiency for all the emitted photons. Typically, L D is extracted by fitting a ratio of the integrated PL of a quenched sample (Q) and an unquenched sample (UQ). This PL ratio reflects the number of recombining excitons (i.e., not collected at the quenching interface) under steady-state: 
    PL^Q/PL^UQ = η _A^Q(1 - η _D^Q)(I_inη _PLη _det)/η _A^UQ(I_inη _PLη _det) = η _A^Q(1 - η _D^Q)/η _A^UQ
 (5) The η A and η D can be simulated using a transfer matrix formalism and a diffusion model as previously described. Here, the SubPc-C 60 PHJ devices in Fig. 1b are used as quenched samples, with C 60 acting as the quencher. A set of unquenched samples ( η D = 0) are fabricated by replacing acceptor C 60 with the exciton blocking material BCP. The resulting PL ratio is plotted in Fig. 3b and fit as a function of SubPc thickness, yielding a SubPc L D of (16.6 ± 2.0) nm. Clearly, the photocurrent-ratio and PL-based measurements conducted on the same set of devices show excellent agreement for the extracted L D . This agreement suggests that the charge recombination present in the device-based measurement does not limit our ability to extract L D . Fig. 3 Photoluminescence-based measurements of exciton diffusion length. a OPVs used for the extraction of L D via photoluminescence (PL) quenching having the structure: ITO/7 nm mCP/X ( = 10–45) nm SubPc/35 nm C 60 (quenched) or BCP (unquenched)/10 nm BCP/1 nm MoO x /100 nm Al. The quenched samples are the same set of devices used for internal quantum efficiency measurements. b PL ratio defined in eq. ( 5 ) versus SubPc thickness. c SubPc PL intensity of the quenched samples versus SubPc thickness. The solid line is fit of the data using eq. ( 4 ). Error bars reflect the run-to-run variation in PL intensity (standard deviation). d Architectures for conventional thin-film PL ratio L D measurements of SubPc and C 60 . SubPc architectures have the structure: glass/10 nm mCP/X ( = 5.0–47.5) nm SubPc/10 nm HATCN (quenched) or mCP (unquenched) while C 60 architectures have the structure: quartz/10 nm BCP/50 nm C 60 /10 nm HATCN (quenched) or BCP (unquenched). e The PL ratio of SubPc films as a function of SubPc thickness. f Excitation spectra (upper panel) for the quenched and unquenched C 60 films at an emission wavelength of 750 nm. The resulting spectrally resolved (SPR) PL ratio versus pump wavelength is shown in lower panel. SubPc films and devices are all pumped with λ = 500 nm light. The incident angle is 70° for all incident light. Error bars for PL ratios are propagated from measured spectra and are proportional to the standard deviation in PL intensity measured multiple times Full size image To further verify the extracted value of L D , we use the L D determined by the PL ratio to simulate the PL of quenched devices with eq. ( 4 ). Figure 3c shows the integrated device PL of SubPc-C 60 PHJ devices as a function of SubPc thickness. Taking the prefactor ( I in η PL η det ) as independent of SubPc thickness, the experimental results are in good agreement with the simulation using L D = 16.6 nm for SubPc. In most reports of PL-based measurements of L D , actual device architectures are not utilized, replaced instead with simple film stacks. In this configuration, exciton dissociation due to bulk-ionization is negligible due to the absence of electrodes. If bulk-ionization in SubPc is negligible for the devices in Fig. 1b , L D values for SubPc extracted from device and thin-film PL should agree. As shown in Fig. 3d , SubPc thin films are deposited on a 10-nm-thick mCP/glass substrate to ensure the SubPc film morphology is similar to the device-based measurement. The quenched films are capped with a 10-nm-thick layer of 1,4,5,8,9,11-hexaazatriphenylene hexacarbonitrile (HATCN) while the unquenched films are capped with a 10-nm-thick layer of mCP [58] . Based on the thickness-dependent PL ratio of Fig. 3e , an intrinsic L D of (16.9 ± 2.0) nm is determined for SubPc. This value is larger than previous reports of the SubPc L D , which is around 10 nm [32] , [59] , [60] . However, previous studies typically deposit SubPc directly on an inorganic substrate such as glass as opposed to a wide energy gap organic buffer layer. By removing the 10-nm-thick mCP layer beneath the SubPc for unquenched samples, we observe a reduction in η PL , suggesting a difference in the morphology of SubPc on different substrates. For weakly luminescent C 60 , a thin layer can result in a very low signal to noise ratio, which increases error for the extraction of L D . As such, we employ a 50-nm-thick C 60 layer and use spectrally resolved (SPR) PL quenching instead of thickness-dependent PL quenching [59] . We also use quartz as the substrate to further reduce the background noise. Figure 3f shows PL excitation spectra for the quenched and unquenched C 60 films at an emission wavelength of λ = 750 nm. The PL ratio is fit as a function of incident excitation wavelength, yielding an intrinsic L D of (18.5 ± 3.0) nm for C 60 . The excellent consistency of results between thin-film and device-based measurements further confirm that an intrinsic L D can be accurately measured using the η IQE -based approach reported here. This agreement also suggests that there are no other diffusive dark states in SubPc and C 60 that contribute to photocurrent since the photocurrent-ratio measurement probes both dark and emissive excitons while the PL-based measurement is only sensitive to emissive states. Relaxation losses for high-energy excited states With the L D of SubPc and C 60 extracted from device photocurrent spectra shown to be intrinsic, materials-relevant quantities, these values can be used to accurately simulate exciton diffusion and recombination losses in OPVs. The unknown geminate recombination loss ( η CS ) that was circumvented in eq. ( 1 ) by taking a ratio of η IQE values can now be calculated as the ratio of η IQE to the calculated η D . 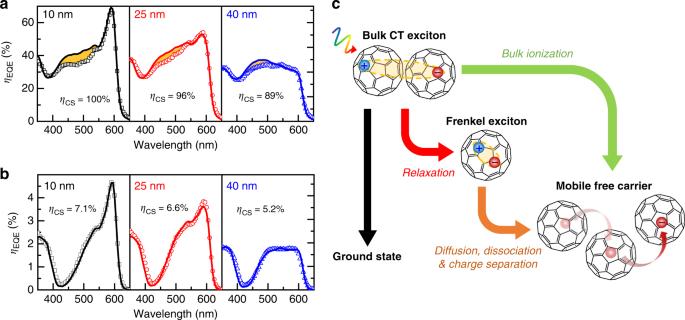Fig. 4 Simulation of external quantum efficiency for extraction of recombination loss.aExternal quantum efficiency spectra for SubPc-C60planar OPVs as a function of SubPc thickness (10, 25, and 40 nm). Experimental results are shown in symbols while solid lines are simulated spectra.bThe experimental (symbols) and simulated (solid lines) external quantum efficiency spectra of SubPc-NPD planar OPVs versus SubPc thickness.cSchematic of free carrier generation in C60from a photoexcited bulk CT exciton. The bulk CT excitons absorb over the wavelength range ofλ= 410 to 550 nm, while the low energy Frenkel excitons correspond to absorption atλgreater than 550 nm Figure 4a shows the simulated η EQE spectra for SubPc-C 60 PHJ devices using the L D extracted in Fig. 1b , and the extracted η CS . The simulated η EQE spectra agree well with experimental results except for the wavelength range of λ = 410–550 nm. The observed η EQE overestimation indicates the presence of a photocurrent loss pathway prior to exciton diffusion, or stated differently, the exciton relaxation yield is not unity. It also worth noting the clear reduction in η CS with increasing donor layer thickness, likely reflecting a reduction in E bi . Fig. 4 Simulation of external quantum efficiency for extraction of recombination loss. a External quantum efficiency spectra for SubPc-C 60 planar OPVs as a function of SubPc thickness (10, 25, and 40 nm). Experimental results are shown in symbols while solid lines are simulated spectra. b The experimental (symbols) and simulated (solid lines) external quantum efficiency spectra of SubPc-NPD planar OPVs versus SubPc thickness. c Schematic of free carrier generation in C 60 from a photoexcited bulk CT exciton. The bulk CT excitons absorb over the wavelength range of λ = 410 to 550 nm, while the low energy Frenkel excitons correspond to absorption at λ greater than 550 nm Full size image To identify whether the exciton relaxation loss is from SubPc or C 60 , a second donor–acceptor system of SubPc-NPD is examined where SubPc serves as the electron acceptor (or hole donor) [7] . To ensure that the SubPc morphology is unchanged, an inverted device architecture is employed (ITO/7 nm mCP/X nm SubPc/35 nm NPD/10 nm mCP/3 nm MoO x /100 nm Al) so that SubPc is still deposited on mCP. In these devices, the electron acceptor SubPc has low electron mobility, which can lead to significant recombination losses due to slow CT state separation [61] . As shown in Supplementary Figure 4 , the SubPc η IQE (from λ = 525 nm) and NPD η IQE (from λ = 385 nm) are both very low (less than 8%). By fitting the η D ratio as a function of SubPc thickness, an L D of (15.2 ± 2.0) nm is obtained for SubPc, close to the value extracted from the SubPc-C 60 system despite significantly increased recombination losses. This result illustrates the power of the photocurrent-ratio technique, even in a low-efficiency device with substantial recombination loss, the correct, intrinsic value of L D is extracted. For the NPD dominant absorption region, an η D (385 nm) = 47.1% is determined. Due to the large spectral overlap between NPD fluorescence and SubPc absorption, the dominant exciton harvesting mechanism within the NPD layer is Förster energy transfer to SubPc instead of exciton diffusion. In order to extract the L D of NPD, a partner material should be chosen with reduced spectral overlap. Figure 4b shows the simulated η EQE spectra for SubPc-NPD PHJ devices based on the parameters extracted. Unlike the SubPc-C 60 case, simulated and experimental η EQE spectra show broadband agreement as a function of SubPc thickness. This suggests that the exciton relaxation losses in SubPc-C 60 devices originate only from excited states in C 60 . Interestingly, the region ( λ = 410–550 nm) where exciton relaxation losses are observed is consistent with the broad absorption peak of C 60 bulk CT excitons [62] . These bulk CT excitons can be photoexcited directly and their absorption ( λ peak around 450 nm) has been observed to decrease drastically when diluting C 60 in thin-film or solution [13] , [63] . This spectral agreement indicates that high energy bulk CT excitons do not uniformly relax to lowest energy Frenkel excitons in C 60 despite their reasonably large energy difference (about 0.5 eV). For the C 60 bulk CT excitons that fail to relax, they may still contribute to photocurrent through bulk-ionization (Fig. 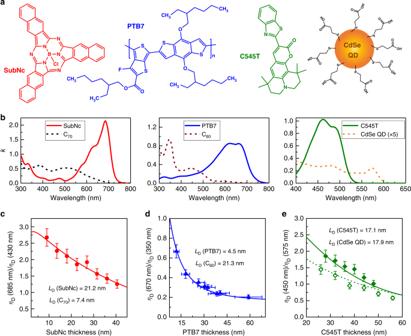Fig. 5 MeasuringLDof dark small molecules, polymers, and quantum dots.aMolecular structure of SubNc, PTB7, C545T and schematic of a CdSe quantum dot (QD) with 3-MPA ligands on the surface.bThe extinction coefficients (k) of SubNc, C70, PTB7, C60, C545T, and CdSe QD thin films. Thekof QDs is shown with a 5-fold magnification.cDiffusion efficiency ratio (λ= 685 nm toλ= 430 nm) as a function of SubNc layer thickness with the corresponding exciton diffusion length (LD) extracted from the fit (solid line) to the data.dDiffusion efficiency ratio (λ= 670 nm toλ= 350 nm) as a function of PTB7 layer thickness.eDiffusion efficiency ratio (λ= 450 nm toλ= 575 nm) as a function of C545T layer thickness and CdSe QD thickness (solid symbols: 66 nm QD layer; open symbols: 42 nm QD layer). TheLDvalues are extracted by fitting both sets of data simultaneously (solid line: fit for 66 nm QD devices; dash line: fit for 42 nm QD devices). Error bars of diffusion efficiency ratio represent run-to-run variation (standard deviation) for the devices tested. Error bars of PTB7 thickness were standard deviation of multiple polymer thin films fabricated with the same procedures 4c ), especially in devices with high built-in fields (see additional discussion in Supplementary Figure 5 , Note 1 ). As such, both relaxation loss and bulk-ionization of bulk CT excitons must be considered in order to accurately simulate broadband η EQE spectra of C 60 -based planar OPVs. Elucidating exciton quenching and dissociation pathways In order to accurately probe intrinsic exciton diffusion in OPVs, the architecture of Fig. 1b was carefully designed to prevent exciton dissociation anywhere but at the D–A interface. As such, comparing its behavior to that of a conventional OPV allows additional exciton dissociation via electrode-organic interfaces and the built-in electric field to be quantified. For instance, removal of mCP between ITO and SubPc (10 nm) leads to a reduction in the SubPc exciton harvesting efficiency, permitting a quantification of quenching at the ITO interface. By inserting a wide gap interlayer to frustrate dissociation at the D–A interface, the photocurrent contribution from bulk-ionization is also quantified. Combining these results with an exciton diffusion model and importantly, accurate measurements of L D , the fraction of photogenerated excitons consumed by various quenching, dissociation, and recombination pathways can be determined, as shown in Supplementary Figure 6 . For λ = 590 nm (mainly SubPc), the fraction of excitons dissociated at the D–A interface, quenched at the ITO-SubPc interface, and undergoing recombination within the donor layer are 73%, 21%, and 6%, respectively. For λ = 450 nm (mainly C 60 ), 88% of C 60 excitons relax to the lowest energy Frenkel states (47% dissociated at D–A interface and 41% recombining in the acceptor layer). Among the remaining 12% bulk CT excitons, 4% can contribute to photocurrent through bulk-ionization and 8% recombine prior to relaxation . These results suggest an important role for bulk-ionization via the built-in-field (especially for bulk CT excitons) in fullerene-based devices. This quantitative decoupling of photoconversion would not be accessible without the device-based L D measurement reported here. Dark small molecules and other excitonic materials With the photocurrent-ratio method thoroughly vetted against conventional PL approaches for SubPc-C 60 , we investigate exciton transport in two dark small molecule materials, boron subnaphthalocyanine chloride (SubNc) and C 70 (Fig. 5a ). While these materials have been frequently utilized in high-efficiency OPVs, their intrinsic L D has not been directly measured as they are inaccessible by PL-based techniques [7] , [12] , [58] , [64] . Similar to the SubPc-C 60 system, we employ a SubNc-C 70 PHJ device with varying donor thickness to extract the intrinsic L D of both dark materials (structure: ITO/8.5 nm mCP/X ( = 9–40.5) nm SubNc/27 nm C 70 /11 nm BCP/1 nm MoO x /100 nm Al). Based on the extinction coefficients (k) of SubNc and C 70 shown in Fig. 5b , the individual η IQE of the donor and acceptor can be extracted from λ = 685 nm (SubNc absorption peak) and λ = 430 nm (primarily C 70 absorption), respectively. By fitting the donor–acceptor η D ratio (determined as previously described) as a function of SubNc thickness (Fig. 5c ), we simultaneously extract an L D of (21.2 ± 2.2) nm for SubNc and an L D of (7.4 ± 0.8) nm for C 70 (see Supplementary Figure 7 for η EQE , η A and η IQE spectra). The longer L D of SubNc compared to SubPc ( L D = 16.7 nm) is consistent with previous observations based on the PL of dilute solid solutions [58] . The extracted L D for C 70 is significantly smaller than that of C 60 ( L D = 18.5 nm). To better understand this difference, further work is needed to investigate differences in exciton lifetime and spin state between these fullerenes. Unlike the SubPc-C 60 case, the simulated broadband η EQE spectra of SubNc-C 70 OPVs agree well with the experimental results, suggesting negligible exciton relaxation loss in C 70 . This result may reflect a reduced CT state character for excitons in C 70 . Fig. 5 Measuring L D of dark small molecules, polymers, and quantum dots. a Molecular structure of SubNc, PTB7, C545T and schematic of a CdSe quantum dot (QD) with 3-MPA ligands on the surface. b The extinction coefficients (k) of SubNc, C 70 , PTB7, C 60 , C545T, and CdSe QD thin films. The k of QDs is shown with a 5-fold magnification. c Diffusion efficiency ratio ( λ = 685 nm to λ = 430 nm) as a function of SubNc layer thickness with the corresponding exciton diffusion length ( L D ) extracted from the fit (solid line) to the data. d Diffusion efficiency ratio ( λ = 670 nm to λ = 350 nm) as a function of PTB7 layer thickness. e Diffusion efficiency ratio ( λ = 450 nm to λ = 575 nm) as a function of C545T layer thickness and CdSe QD thickness (solid symbols: 66 nm QD layer; open symbols: 42 nm QD layer). The L D values are extracted by fitting both sets of data simultaneously (solid line: fit for 66 nm QD devices; dash line: fit for 42 nm QD devices). Error bars of diffusion efficiency ratio represent run-to-run variation (standard deviation) for the devices tested. Error bars of PTB7 thickness were standard deviation of multiple polymer thin films fabricated with the same procedures Full size image To demonstrate the applicability of the photocurrent-ratio method in other excitonic systems, we also show two examples measuring exciton transport in solution processed PTB7 polymer films and inorganic CdSe quantum dot (QD) films. PTB7 is a high-performing polymer electron donor in OPVs, with demonstrated power efficiencies as high as 9.2% when combined with the fullerene acceptor PC 71 BM [65] . Here, we employ it as an electron-donor material paired with fullerene acceptor C 60 . Figure 5d shows the PTB7-C 60 η D ratio as a function of PTB7 thickness obtained from planar OPVs with a structure: ITO/2.5 nm HfO 2 /X ( = 12–59) nm PTB7/37 nm C 60 /10 nm BCP/1 nm MoO x /100 nm Al (see Supplementary Figure 8 for η EQE , η A and η IQE spectra). A thin layer of wide energy gap HfO 2 is utilized as an exciton blocking layer at ITO/donor interface (deposited via atomic layer deposition). The donor η IQE is extracted from λ = 670 nm (PTB7 absorption peak) while the acceptor η IQE is extracted from λ = 350 nm (C 60 Frenkel exciton absorption peak). As negligible exciton relaxation loss is observed at λ = 350 nm in the previous SubPc-C 60 case (Fig. 4a ), it is assumed that C 60 has 100% exciton relaxation yield at this wavelength. Fitting the η D ratio in Fig. 5d yields a short L D of (4.5 ± 0.5) nm for PTB7 and an L D of (21.3 ± 2.2) nm for C 60 . The C 60 L D is similar to the value extracted from the SubPc-C 60 system (18.5 nm). For CdSe QD thin films, the QDs are zincblende nanocrystals (size ~4 nm) stabilized with 3-mercaptopropionic acid (3-MPA) after treatment via solid-state ligand exchange [66] . The resulting thin films have a very low extinction coefficient (k = 0.05 at excitonic peak, λ = 575 nm), and are therefore paired with a wider energy gap small molecule 2,3,6,7-tetrahydro-1,1,7,7,-tetramethyl-1H,5 H,11H-10-(2-benzothiazolyl)quinolizino[9,9a,1gh]coumarin (C545T), which does not absorb at λ = 575 nm. Wide gap materials HfO 2 and di-[4-(N,N-di-p-tolyl-amino)-phenyl]cyclohexane (TAPC) are utilized as exciton blocking layers for CdSe QDs and C545T, respectively. The CdSe QD-C545T planar cell has an inverted device architecture: ITO/2.5 nm HfO 2 /X (= 42, 66) nm CdSe QD/Y ( = 26–56) nm C545T/11 nm TAPC/10 nm MoO x /100 nm Al, where the CdSe QDs serves as the electron acceptor layer and photogenerated electrons are collected at ITO. It is again worth noting the ability of the photocurrent-ratio method in yielding intrinsic values of L D even in devices with low efficiency. This allows active materials to be selected solely on the basis of realizing a minimal overlap in optical absorption. The QD film thickness is controlled by the number of cycles for the ligand exchange process [66] . Figure 5e shows the C545T-CdSe QD η D ratio as a function of C545T thickness for two different QD film thicknesses (see Supplementary Figure 9 for broadband η EQE , η A and η IQE spectra). The donor η IQE is extracted at λ = 450 nm (C545T absorption peak) while the acceptor η IQE is extracted at λ = 575 nm (QD excitonic absorption peak). Results for devices with QD layer thickness of 42 nm and 66 nm are fitted simultaneously, yielding an L D of (17.9 ± 3.6) nm for the CdSe QDs and an L D of (17.1 ± 3.4) nm for C545T. It is worth noting that the L D of C545T extracted here is consistent with separate PL-based measurements we have carried out (16.7 nm). If instead the η D ratio is fit for each QD thickness, the 42 nm (66 nm) QD-C545T devices yield an L D of 18.7 nm (15.5 nm) and 19.8 nm (16.8 nm) for the QDs and C545T, respectively. The L D of CdSe QDs extracted here is smaller than that previously reported for CdSe core-shell counterparts (20 to 40 nm) [67] , [68] , likely reflecting that a wide gap shell is critical to frustrate exciton decay and enhance exciton transport for CdSe QDs. We demonstrate a simple photocurrent-ratio method to measure the intrinsic L D of excitonic semiconductors in bilayer photovoltaic cells. The impact of often unknown recombination losses is negated when taking a ratio of donor and acceptor η IQE . For the luminescent organic pairing SubPc and C 60 , their L D extracted using this method are in excellent agreement with those extracted from conventional PL-quenching measurements, a direct result of the ability to remove the role of unknown geminate recombination losses. With knowledge of the intrinsic values of L D , we are able to investigate the potential for relaxation losses, which are typically overlooked in device-based studies of L D . Indeed, bulk CT excitons generated in C 60 have non-unity relaxation yield to Frenkel states and can generate free carriers directly through bulk-ionization. The generality of this photocurrent-ratio method is further demonstrated by extracting L D for the dark small molecule SubNc, C 70 , the high-performance polymer PTB7, as well as for CdSe quantum dot thin films. Thus, we demonstrate a straightforward measurement for the extraction of L D that is equally applicable to both luminescent and dark excitonic materials capable of being integrated into a bilayer photovoltaic cell. Chemicals For this study, SubPc (99%), mCP (99%), TPBi (99%), C545T (99%), TAPC (99%), and PTB7 (Mw > 50,000) were obtained from Lumtec Inc., C 60 (99%) and C 70 (99%) were obtained from MER Corporation, MoO 3 (99%) and BCP (98%) were obtained from Alfa Aesar, chloroform (99%), 3-mercaptopropionic acid (99%), octane (98%), oleic acid (tech. grade 90%) acetonitrile (99.5%), and methyl acetate (anhydrous) were obtained from Sigma–Aldrich, selenium dioxide (99.8%) and 1-octadecene (90%) were obtained from Acros Organics. All materials above were used as received. The NPD (99%) was synthesized by the Dow Chemical Company and purified once by temperature-gradient sublimation [69] . Cadmium myristate was prepared on a multi-gram scale according to the method reported by Chen et al. [70] . Synthesis of zincblende CdSe QDs Zincblende CdSe QDs with oleic acid capping ligands were synthesized as previously reported [66] , based off the original synthesis by Chen and et al. [70] . Briefly, 1-octadecene (63 mL), cadmium myristate (570 mg) and selenium dioxide (110 mg) were added to a 3-neck round bottom flask and degassed at 75 °C for 1 h. After degassing, the reaction mixture was heated to 240 °C, at which point 1 mL of oleic acid was added dropwise to the solution once a red color was achieved. The reaction was allowed to proceed for 15 min and then cooled to room temperature for purification by centrifugation in methyl acetate. The resulting precipitate was dispersed in octane and filtered using a 0.2 um PTFE syringe filter prior to film fabrication. Resulting solution concentration was ~25 g L −1 . Thin-film and device preparation Organic photovoltaic cells were fabricated using indium-tin-oxide (ITO)-coated glass substrates with a sheet resistance of 8–12 Ω per □. Substrates were cleaned in tergitol solution and in organic solvents and treated in UV-Ozone ambient for 10 min prior to thin-film deposition. All polymer and QD films were spin-coated onto an HfO 2 -coated ITO substrate. The HfO 2 was deposited via atomic layer deposition at 200 °C. The polymer PTB7 was first dispersed in chloroform and then spin-coated at 3000 rpm for 45 s. The obtained samples were annealed in N 2 at 140 °C for 10 min. The polymer film thickness was controlled via the concentration of the PTB7 solution (2–10 g L −1 ). Spin-coating and buildup of QD film thickness were realized using a solid-state ligand exchange procedure. CdSe QDs dispersed in octane were spin-coated at 1200 rpm for 30 s and then 6000 rpm for 60 s. The latter process is found to improve film uniformity and reproducibility. Next, 3-MPA (1% v/v) in acetonitrile was first deposited onto the film and allowed to sit for 10 s to facilitate the ligand exchange. The sample was then spun again at 1200 rpm for 30 s. Finally, the film was rinsed with pure acetonitrile by spinning at 6000 rpm for 60 s. This process was repeated 3–4 times until the desired QD film thickness was achieved. All other layers were deposited at room temperature by high vacuum thermal evaporation at a pressure of less than 8 × 10 –7 Torr. The active area of the obtained device is 0.785 mm 2 , defined by the cathode area. Optoelectronic characterization Photoluminescence quenching data were recorded using a Photon Technology International QuantaMaster Fluorometer. All photoluminescence measurements were performed under N 2 purge. Photoluminescence quenching measurements were made at an incident angle of 70° to the substrate normal. External quantum efficiency measurements were collected by measuring the photocurrent under monochromatic light illumination using a 300 W Oriel Xe lamp, a monochromator, an optical chopper wheel, and an SR810 lock-in amplifier. Error bars for L D represent a 95% confidence interval extracted from fitting parameters. All film thicknesses, reflectivity spectra were measured with a J. A. Woollam spectroscopic ellipsometer. The device reflectivity measurements were made at an incident angle of 15° to the substrate normal. Film thicknesses were fit using a Cauchy model. For simulations of device absorption efficiency optical constants of organic and QD thin films were extracted by fitting transmission (at normal incidence) and reflection (incident angle: 15°) simultaneously with a transfer matrix formalism (provided in Supplementary Figure 10 ).